Polymeric molecular sieve membranes viain situcross-linking of non-porous polymer membrane templates High-performance polymeric membranes for gas separation are attractive for molecular-level separations in industrial-scale chemical, energyand environmental processes. Molecular sieving materials are widely regarded as the next-generation membranes to simultaneously achieve high permeability and selectivity. However, most polymeric molecular sieve membranes are based on a few solution-processable polymers such as polymers of intrinsic microporosity. Here we report an in situ cross-linking strategy for the preparation of polymeric molecular sieve membranes with hierarchical and tailorable porosity. These membranes demonstrate exceptional performance as molecular sieves with high gas permeabilities and selectivities for smaller gas molecules, such as carbon dioxide and oxygen, over larger molecules such as nitrogen. Hence, these membranes have potential for large-scale gas separations of commercial and environmental relevance. Moreover, this strategy could provide a possible alternative to ‘classical’ methods for the preparation of porous membranes and, in some cases, the only viable synthetic route towards certain membranes. Membrane-separation technology has become a promising alternative to conventional energy-intensive separation processes such as distillation or absorption in a variety of applications including natural gas sweetening, hydrogen recovery and production, carbon dioxide separation from flue gas and air separation [1] . Over the past decade, significant progress has been made in molecular sieving materials such as zeolites [2] , [3] , silica [4] , metal organic frameworks [5] and carbon-based membranes [6] , [7] , [8] . However, it is often difficult to both process these materials into membranes and functionalize the micropores, which has limited their gas-separation properties and further hindered the development of this field. Furthermore, membranes based on such microporous materials have not found commercial applications in gas separation because of scale-up impracticalities and high cost [9] . Polymer membranes provide an energy-efficient method of gas separation because they do not require thermal regeneration, a phase change or active moving parts in their operation; therefore, they are expected to play a growing role in an energy-constrained and low-carbon future [10] , [11] , [12] , [13] , [14] , [15] . Most commercial polymer membranes for gas separation have been limited to a small number of polymers with low permeability and high selectivity, creating the need for large areas to compensate for the lack of permeance. This increases both costs and space requirements for large-scale applications [16] , [17] . Microporous polymers with high permeability demonstrate insufficient selectivity for practical applications, because they possess ill-defined voids that fluctuate in size because of chain flexibility that effectively limits size selectivity [18] . Moreover, the fact that most microporous polymers are synthesized in powder form and are insoluble in solvents makes the adaptation of this methodology to the preparation of membranes extremely difficult. Therefore, it remains a great challenge to develop a general, effective approach for preparing porous polymeric membranes that behave as efficient molecular sieves, so that they provide both the permeability and selectivity needed to support large-scale gas separations. Recently, covalently linked microporous organic polymers (MOPs) have attracted considerable attention because their structures and properties can be easily modified through rational chemical design and synthesis [19] . A number of MOPs have been synthesized through various coupling reactions including crystalline polymers such as covalent organic frameworks, amorphous polymers such as polymers of intrinsic microporosity and conjugated microporous polymers [20] , [21] , [22] , [23] , [24] , [25] , [26] , [27] . Hypercross-linked polymers represent a new class of porous materials that are prepared mainly by a Friedel–Crafts alkylation reaction [28] , [29] , [30] . The permanent porosity in hypercross-linked polymers is a result of extensive cross-linking reactions, which prevent the polymer chains from collapsing into a dense, non-porous state [31] , [32] , [33] . Herein we describe a facile, versatile, yet unexplored approach, referred to as an in situ cross-linking strategy, for the preparation of polymeric molecular sieve membranes having a sandwich structure with hierarchical and tailorable porosity. The structure comprises a macroporous core, a layer of dense micropores and a mesoporous surface composed of small polymer nanoparticles. The process uses non-porous polystyrene (PS) membranes as a precursor membrane template ( Fig. 1a ). Then, based on the Friedel–Crafts reaction, PS membranes are readily cross-linked in situ to produce hypercross-linked porous polymeric membranes. In the cross-linking process, formaldehyde dimethylacetal (FDA) is used as a cross-linker and FeCl 3 as a catalyst. This synthesis offers both tunable porosity and the formation of three well-defined pore networks, and these characteristics make our new membranes amenable to quantitative modelling of their mass transport properties. Thus, the porous polymeric membranes obtained exhibit properties that are promising for use in gas separations with high permeability and favourable selectivity, and they show great potential for prospective applications in liquid separations and membrane catalysis. 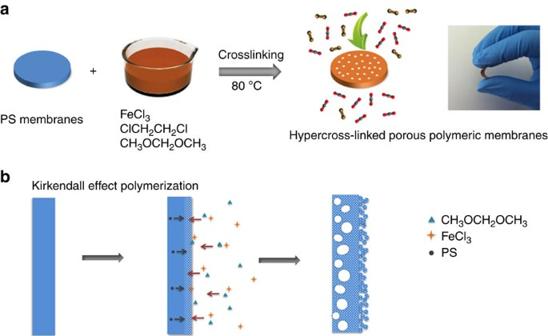Figure 1: Synthesis of the hypercross-linked porous polymeric membranes. Schematic illustration of (a) the preparation procedure for the porous polymeric membranes and (b) the non-equilibrium diffusion at the interface in membrane by Kirkendall effect polymerization (the reaction is only shown for one side of the membrane). Figure 1: Synthesis of the hypercross-linked porous polymeric membranes. Schematic illustration of ( a ) the preparation procedure for the porous polymeric membranes and ( b ) the non-equilibrium diffusion at the interface in membrane by Kirkendall effect polymerization (the reaction is only shown for one side of the membrane). Full size image Synthetic approach and characterization of the porous membranes PS is a common commercial polymer that is easily fabricated into membranes by dissolution in a nonpolar solvent and casting on a suitable substrate. By simply immersing the non-porous PS membranes in a mixture of the cross-linker FDA, the catalyst FeCl 3 , and the solvent 1, 2-dichloroethane the PS membranes could be readily cross-linked when heated to 80 °C. The resulting membranes were washed with acetone, dilute hydrochloric acid and deionized water, and then dried in a vacuum oven at 60 °C. The cross-linked membranes were completely insoluble in common organic solvents such as chloroform and toluene. The dimension and shape of the cross-linked membranes were essentially determined by those of the precursor PS membranes. The morphology and nanostructure of the membranes were characterized by scanning electron microscopy (SEM), transmission electron microscopy (TEM) and atomic force microscopy (AFM). A smooth, defect-free PS membrane surface and non-porous structure were revealed by AFM and SEM. ( Supplementary Fig. 1 ). Even after a cross-link time of 24 h, the membranes remained flexible and continuous without any noticeable pinholes or cracks at the micrometre scale ( Figs 1a and 2a,b ). The polymeric membranes produced have thicknesses of ~86, 97 and 109 μm, depending on the initial thickness of the PS membranes— ~50, 65 and 85 μm. As the three cross-linked membranes have similar characterization results ( Fig. 2 and Supplementary Figs 2 and 3 ), we will focus our discussion on the 97-μm membrane since we consider it to be representative of all the three membranes. Remarkably enough, the top view and the cross-sectional SEM and high-resolution TEM images of the 97-μm membrane clearly reveal the sandwich structure with hierarchical porosity comprising a macroporous core, a layer of dense micropores and a mesoporous surface. The observations with the SEM at higher magnification and with the AFM show that the outer continuous network of the mesoporous surface is composed of small polymer nanoparticles with 15–30 nm diameters ( Fig. 2a,b ). Closer examination of the mesopores on the cross-section of the membrane reveals that the mesopores run from the top surface into the underlying microporous layer, and the thickness of the mesoporous layer is ~1 μm ( Fig. 2d ). Randomly distributed macroporosity is observed on the micrometre-length scale throughout the interior of the membrane ( Fig. 2c and Supplementary Fig. 4 ). These macropores, albeit broadly distributed in size (500 nm–3 μm), form an interconnected network characteristic of co-continuous structures. Within the entire polymer membrane struts, a large number of micropores with a pore size of 0.5 nm can be observed, as estimated from an analysis of the high-resolution TEM images, and a fraction of the pores are accessible from the mesopores and macropores ( Fig. 2e,f and Supplementary Fig. 4 ). In addition, the tensile strains at break are 3.56, 15.75 and 31.91%, while the tensile stresses at break are 1.38, 3.45 and 9.01 MPa for the porous membranes with different thicknesses of 109, 97 and 86 μm, respectively ( Supplementary Table 1 ). 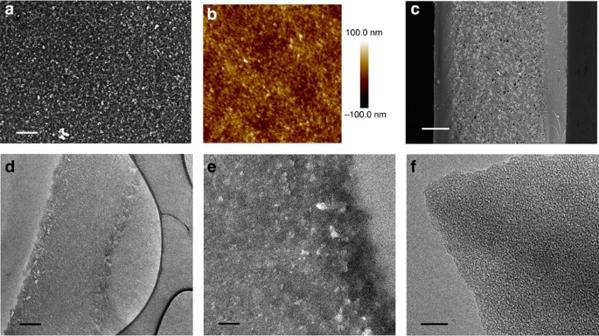Figure 2: Electron microscopy characterization of the porous polymeric membranes. SEM images of the 97-μm porous polymeric membranes cross-linked for 24 h: top view (a; scale bar, 500 nm) and cross-section (c; scale bar, 20 μm). AFM (4 × 4 μm2;b) and high-resolution TEM images (d–f) of this porous membrane (scale bars, 200, 50 and 10 nm, respectively). Figure 2: Electron microscopy characterization of the porous polymeric membranes. SEM images of the 97-μm porous polymeric membranes cross-linked for 24 h: top view ( a ; scale bar, 500 nm) and cross-section ( c ; scale bar, 20 μm). AFM (4 × 4 μm 2 ; b ) and high-resolution TEM images ( d – f ) of this porous membrane (scale bars, 200, 50 and 10 nm, respectively). Full size image The structural properties of the porous polymeric membranes were characterized using various spectroscopic measurements and thermogravimetric analysis. The improved stability of the cross-linked porous membrane, relative to the precursor, is consistent with the generation of a rigid cross-linking polymeric framework ( Supplementary Fig. 5a ). The Fourier transform infrared spectra of the cross-linked membrane show bands at ~1,600, 1,500 and 1,440 cm −1 that can be attributed to aromatic ring skeleton vibrations consistent with the structure of PS ( Supplementary Fig. 5b ). A band at 1,693 cm −1 due to C=O stretching vibration was observed. We hypothesize that during the cross-linking process, some of the cross-linker molecules react with only one benzene ring owing to steric hindrance and subsequently become further oxidized to C=O groups by the Fe 3+ catalyst. Solid-state 13 C cross-polarization magic angle spinning nuclear magnetic resonance spectroscopy shows resonance peaks near 137 and 130 p.p.m., which are assigned to aromatic carbon and non-substituted aromatic carbon, respectively. The resonance peak near 43 p.p.m. could be assigned to the carbon in the methylene linker formed after Friedel–Crafts reaction [30] . The resonance peaks between 150 and 200 p.p.m. further confirm the formation of the C=O group ( Fig. 3a ). From the elemental analysis, the porous membranes are composed of C 90.98 wt%, H 7.2 wt% and O (calculated) 1.82 wt%. Energy-dispersive X-ray spectroscopy results show that about 2% iron still remain in the membrane after washing several times with different solvents ( Supplementary Fig. 6 ). 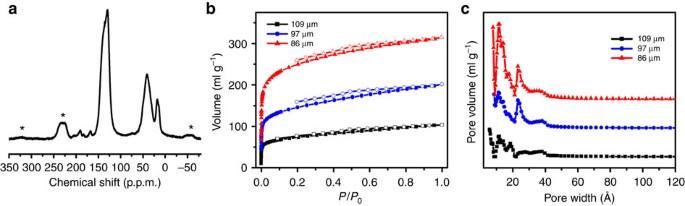Figure 3: Structure and porosity characterization of the porous polymeric membranes. (a) Cross-polarization (CP)13C MAS natural abundance NMR spectrum of the 97-μm porous polymeric membrane. Asterisks denote spinning sidebands. (b,c) Nitrogen adsorption–desorption isotherms at 77 K and pore size distributions based on non-local density functional theory (NLDFT) calculation for the porous membranes with different thicknesses. Figure 3: Structure and porosity characterization of the porous polymeric membranes. ( a ) Cross-polarization (CP) 13 C MAS natural abundance NMR spectrum of the 97-μm porous polymeric membrane. Asterisks denote spinning sidebands. ( b , c ) Nitrogen adsorption–desorption isotherms at 77 K and pore size distributions based on non-local density functional theory (NLDFT) calculation for the porous membranes with different thicknesses. Full size image The pore structure of the membranes was investigated by nitrogen sorption analysis measured at 77 K. The N 2 adsorption–desorption isotherms of porous polymeric membranes with different thicknesses exhibit a type I reversible sorption profile with a slight hysteresis loop at higher relative pressures, indicating abundant micropore structure and the presence of mesopores in the membrane surface ( Fig. 3b ). The controllable surface areas of the porous membranes range from 260 to 792 m 2 g −1 , increasing as the membrane thickness decreases from 109 to 86 μm. As the in situ cross-linking process begins at the surface and continues to the interior of the PS membranes, it proceeds more easily in the thinner membranes owing to faster mass transport, which results in a higher surface area. Therefore, the thickness of the initial PS membranes has a dramatic effect on the surface areas of the final porous membranes. In addition, all the membranes exhibit a similar pore size distribution with a dominant pore size of 5.1 Å ( Fig. 3c ) as calculated using non-local density functional theory in good agreement with the size range obtained from high-resolution TEM images. Moreover, the mesopore sizes are in the range of 2–4.4 nm in these membranes. The pore size distribution curves suggest that all the membranes have hierarchical porosity and are predominantly microporous. Gas separation properties of the porous polymeric membranes Given the hierarchical porous structures and excellent surface areas, the gas-separation capabilities of the porous polymeric membranes were examined using a non-steady-state permeation cell at a temperature of 298 K and a pressure difference of 0.35 bar. The CO 2 permeabilities and ideal selectivities of the porous polymeric membranes of varying thickness (86–109 μm) are given in Table 1 . The CO 2 permeabilities of the membranes are particularly high, which is consistent with their enhanced hierarchical porosity and high surface areas. Under the same test condition, the CO 2 flux through the PS membranes was below the detection limit of the instrument and was not measured because of the non-porous structure. As the thickness of the porous polymeric membranes decreases from 109 to 86 μm, CO 2 permeabilities increase greatly, from 117 to 26,756 barrer and selectivities decrease from 27.1 to 7. Polymeric membranes generally suffer from a well-defined trade-off between the properties of permeability and selectivity [34] , [35] . This is typically illustrated using a plot of selectivity versus permeability, generally called a Robeson plot, and is shown in Fig. 4a . The membrane with a thickness of 97 μm demonstrates both excellent permeability and selectivity, as shown by its position at the Robeson upper bound for CO 2 /N 2 gas pairs. The membranes were tested through six cycles under the same conditions and exhibited minimal change in either CO 2 permeability or CO 2 /N 2 selectivity, indicating that the membranes are a stable system suitable for CO 2 sequestration. It is important to note that only carbon and hydrogen form the polymeric framework with no other elements or functional groups improving the gas adsorption and diffusion during the separation process. Therefore, the membrane performance can be directly ascribed to the molecular sieving characteristics of the membranes, which facilitate enhanced diffusivity and selectivity for CO 2 molecules with a smaller kinetic diameter (CO 2 =3.3 Å) compared with N 2 molecules having a larger diameter (N 2 =3.64 Å). The hierarchical pore structure enables more rapid diffusion of gas molecules through these polymeric membranes as compared with traditional gas-separation membranes while the abundant microporosity throughout the polymeric framework leads to effective gas separation. The combination of the two factors results in the high permeability and excellent selectivity of the porous polymeric membranes. Table 1 Permeability and ideal selectivity values for porous polymeric membranes. 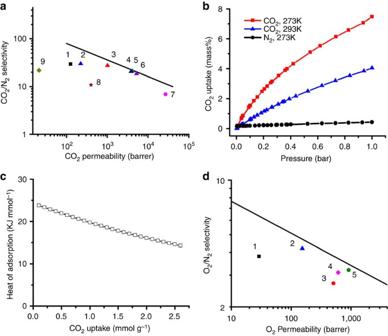Figure 4: Gas separation performance of the porous polymeric membranes. (a) The Robeson plot relevant to porous polymeric membranes for a CO2/N2gas pair showing the data for the 109, 97 and 86 μm membranes cross-linked for 24 h (1, 6, 7); the 97 μm membranes cross-linked for 1.5, 3, 6 and 12 h (2–5); and the cross-linked PS-PB-PS (8) and PS-PEB-PS (9) membranes. (b) CO2and N2adsorption isotherms of the 97-μm porous membranes cross-linked for 24 h measured at 273 and 298 K. (c) Isosteric heats of adsorption for the porous membranes at different CO2loadings. (d) The Robeson plot relevant to porous membranes for O2/N2showing the data for the 97-μm membranes cross-linked for 1.5, 3, 6, 12 and 24 h (1–5). Full size table Figure 4: Gas separation performance of the porous polymeric membranes. ( a ) The Robeson plot relevant to porous polymeric membranes for a CO 2 /N 2 gas pair showing the data for the 109, 97 and 86 μm membranes cross-linked for 24 h (1, 6, 7); the 97 μm membranes cross-linked for 1.5, 3, 6 and 12 h (2–5); and the cross-linked PS-PB-PS (8) and PS-PEB-PS (9) membranes. ( b ) CO 2 and N 2 adsorption isotherms of the 97-μm porous membranes cross-linked for 24 h measured at 273 and 298 K. ( c ) Isosteric heats of adsorption for the porous membranes at different CO 2 loadings. ( d ) The Robeson plot relevant to porous membranes for O 2 /N 2 showing the data for the 97-μm membranes cross-linked for 1.5, 3, 6, 12 and 24 h (1–5). Full size image To provide a better understanding of the membrane-separation performance, the CO 2 adsorption of a 97-μm membrane was measured up to 1 bar at 273 K using a gravimetric microbalance (IGA, Hiden Isochema) and was shown to be 1.70 mmol g −1 (7.47 mass%; Fig. 4b ). The N 2 uptake of this sample under the same conditions was 0.154 mmol g −1 (0.431 mass%). The estimated CO 2 /N 2 adsorption selectivity was ~40. By fitting the CO 2 adsorption isotherms measured from 0.001 to 1 bar at different temperatures (273 and 298 K) and applying a variant of the Clausius–Claperyron equation, we calculated the isosteric heat of adsorption to be in the range 14.3–23.8 kJ mol −1 , much smaller than those of common MOP materials (25–33 kJ mol −1 ). This further confirms that the molecular sieving effect is responsible for the extraordinary membrane-separation performance ( Fig. 4c ) [36] . Adjusting the cross-linking time One of the important advantages of the porous polymeric membranes is the versatility and flexibility in precisely tailoring the structure and gas-separation performance, which can be tuned by simply adjusting the cross-linking time. 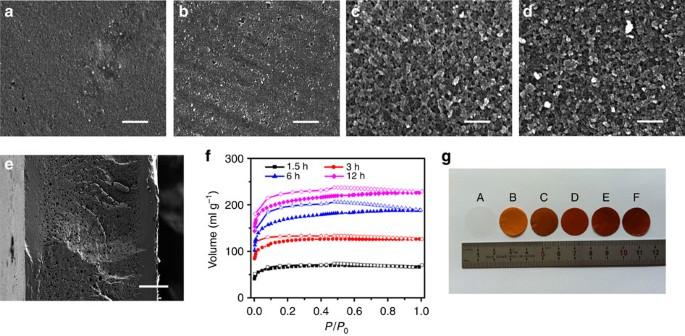Figure 5: Characterization of the membranes with different cross-linking times. Top-view SEM images of the 97-μm porous polymeric membranes cross-linked for (a) 1.5 h, (b) 3 h, (c) 6 h and (d) 12 h (scale bars, 500 nm). (e) Cross-sectional SEM image of the membrane cross-linked for 1.5 h (scale bar, 20 μm). (f) N2adsorption–desorption isotherms of the porous membranes cross-linked for different times. The isotherm is offset vertically by 40 ml g−1ford. (g) PS membrane (a) and porous membranes cross-linked for 1.5 (b), 3 (c), 6 (d), 12 (e) and 24 h (f). Figure 5a–d show SEM micrographs of the top view of membranes of the same thickness (97 μm) reacted under identical conditions but with different cross-linking times of 1.5, 3, 6 and 12 h. These micrographs elucidate the membrane surface structure dependence on the length of the cross-linking step. After short cross-linking times (that is, 1.5 and 3 h), the membranes have a dense microporous skin layer, but only a few mesopores are beginning to nucleate at the surface. Increasing the cross-linking time to 6–24 h produced the desired open network nanostructure, that is, a selective skin layer containing a high density of mesopores 12~50 nm in diameter randomly distributed across the surface. As the cross-linking time is further increased, the surface mesopores increase in size and the membrane becomes more open, whereas the interior macropore layer does not change significantly ( Fig. 5e and Supplementary Fig. 7 ). All the isotherms of the porous membranes with various cross-linking times also exhibit characteristic type I curves with distinct capillary condensation steps suggesting uniform micropores. The surface areas increase from 218 to 618 m 2 g −1 with the increase in cross-linking time ( Fig. 5f ). After a cross-link time of 6–24 h, the membranes show a similar surface area of 593±36 m 2 g −1 and pore volume of 0.283±0.015 cm 3 g −1 , which clearly indicates that the cross-linking process between FDA and PS membranes happens very fast, and could even completely finish within 6 h. Furthermore, as the cross-linking time increases, the CO 2 permeabilities increase from 222.2 to 5261 barrer, and CO 2 /N 2 selectivities decrease from 30 to 18.5 ( Table 1 and Fig. 4a ). Therefore, adjusting the cross-linking time can produce polymeric membranes with desirable pore structures, surface areas and commercially favourable gas-separation performance. In addition, sheets of 97 μm membranes as large as 100 cm 2 were fabricated in the laboratory for gas-separation testing, indicating that this method has the important advantage of industrial scalability. Figure 5: Characterization of the membranes with different cross-linking times. Top-view SEM images of the 97-μm porous polymeric membranes cross-linked for ( a ) 1.5 h, ( b ) 3 h, ( c ) 6 h and ( d ) 12 h (scale bars, 500 nm). ( e ) Cross-sectional SEM image of the membrane cross-linked for 1.5 h (scale bar, 20 μm). ( f ) N 2 adsorption–desorption isotherms of the porous membranes cross-linked for different times. The isotherm is offset vertically by 40 ml g −1 for d . ( g ) PS membrane ( a ) and porous membranes cross-linked for 1.5 ( b ), 3 ( c ), 6 ( d ), 12 ( e ) and 24 h ( f ). Full size image O 2 /N 2 separation Separation of O 2 /N 2 is an important process that has been applied on an industrial scale for applications such as O 2 enrichment from air (medical devices) and N 2 enrichment from air (used to protect the atmosphere for oxygen-sensitive compounds) [37] . As they have nearly identical kinetic diameters, the O 2 /N 2 separation process is much more difficult to achieve compared with many other gas pairs. The porous polymeric membranes also show promise for the separation of O 2 from N 2 , as their permeability data are close to the Robeson upper bound ( Fig. 4d ). As with CO 2 /N 2 pairs, the O 2 /N 2 selectivities decrease from 4.2 to 3.1 as the cross-linking time increases, whereas the O 2 permeabilities increase from 29.1 to 222.2 barrer. This exceptional O 2 /N 2 separation performance is similar to the performance of carbon molecular sieve membranes, further indicating that the gas-separation performance of the porous membranes is due to a molecular sieving effect [38] , [39] , [40] . This result suggests that these porous membranes have excellent potential for the important industrial applications of N 2 and O 2 enrichment from air. Cross-linking other PS-based membranes This in situ cross-linking method can be extended to cross-link other PS-based block polymer membranes to prepare functionalized porous membranes. The surface area and pore volume of cross-linked PS-block-polybutadiene-block-PS (PS-PB-PS) membranes are 209 m 2 g −1 and 0.11 cm 3 g −1 , respectively, clearly indicating that the flexible polybutadiene chains increase framework density and may block some parts of the micropores ( Supplementary Fig. 8c ). The CO 2 permeability and CO 2 /N 2 selectivity were measured at 398 barrer and 10.9, respectively ( Table 1 and Fig. 4a ). Although no surface area could be measured by nitrogen sorption analysis for cross-linked PS-block-poly(ethylene-ran-butylene)-block-PS-graft-maleic anhydride (PS-PEB-PS) membranes, CO 2 permeability and CO 2 /N 2 selectivity were still 21.3 and 21.8, respectively ( Table 1 and Fig. 4a ). This indicates the presence of ultra-small micropores in the framework of the cross-linked membrane that allow only the smaller diameter CO 2 molecules to pass through. SEM images of these two cross-linked polymeric membranes reveal their dense structures, which further confirm that such a hierarchical porous structure greatly accelerates the gas diffusion rate during the separation process and simultaneously maintains high selectivity ( Supplementary Fig. 8a,b,d,e ). Furthermore, the cross-linked PS-PEB-PS membranes are flexible and stretchable and could even be rolled up ( Supplementary Fig. 8f,g ). The tensile strains at break are 36.58 and 29.96%, while the tensile stresses at break are 11.72 and 20.02 MPa for the cross-linked PS-PB-PS and PS-PEB-PS membranes ( Supplementary Table 1 ). On the basis of these observations, we propose a one-pot polymerization-induced Kirkendall effect mechanism for the formation of sandwich-structured polymeric molecular sieve membranes with hierarchical porosity ( Fig. 1b ) [41] , [42] . The PS membrane surface first reacts very fast with FDA to produce a layer consisting of a microporous cross-linked polymer shell. The cross-linked layer is stable and insoluble in 1, 2-dichloroethane. The direct conversion of PS to porous polymer and the dissolution of interior PS are therefore hindered by the layer and the reaction will continue by the diffusion of FDA and FeCl 3 through the microporous layer. During this step, the diffusion rate of PS is faster than those of FDA and FeCl 3 . The preferred outward diffusion of PS molecules from core to shell leads to a net material flux across the membrane interface and simultaneously results in a flow of fast-moving vacancies to the vicinity of the solid–liquid interface. The macroporous core is formed through coalescence of the vacancies based on a nanoscale Kirkendall effect. With an increased degree of cross-linking, the surface micropores can gradually transform into mesopores and the mesopores can increase in size. In situ cross-linking on the interfaces facing towards both the shell region and the core region yields fully microporous skeletal networks throughout the membrane thickness, forming a sandwich structure with a multiscale tricontinuous network through which gases can be easily transported and effectively separated. In summary, we develop a facile, versatile one-pot approach for the preparation of hierarchically macro-, meso- and microporous polymeric molecular sieve membranes via in situ cross-linking of PS membranes, and introduce techniques for their quantitative structural characterization. The porous membranes exhibit promising properties for use in gas separations, demonstrating both excellent permeability and selectivity. Specifically, the tunable structural characteristics, adjustable gas-separation properties and controllable chemical functionalities of this system provide an exceptional platform for the fabrication of polymeric gas-separation membranes. Furthermore, given the range of available polymer species, the in situ cross-linking method can be extended to prepare other types of polymer membranes with desired properties, and we anticipate that this study will expand the viability of such porous membranes to a wide variety of fields. Fabrication of PS membrane PS (Mw ca. 15,900) was dissolved in toluene or CH 2 Cl 2 to from 16.7 and 28.6 wt% polymer solutions. These solutions were then drawn into a membrane on a glass substrate using a doctors blade set at a gate height of 254 or 381 μm. After the membranes were cast, the solvent was allowed to evaporate for a predetermined period of time. Finally, PS membranes of varying thickness were successfully fabricated. The membranes derived from different PS molecular weights (Mw ca. 35,000 and 192,000), PS-PB-PS (styrene 30 wt %, Mw ca. 140,000) and PS-PEB-PS (styrene 22 wt%, Mw ca. 128,000) were fabricated by the same method. Synthesis of porous polymeric membrane FeCl 3 (4.875 g, 0.03 mol), FDA (2.28 g, 0.03 mol) and 10 ml 1, 2-dichloroethane were combined and stirred in an ice bath until completely mixed. Several pieces of PS membranes were added to the mixture, and then the mixture was heated to 80 °C for 24 h without stirring. The resulting membranes were washed with acetone, 1 M hydrochloric acid and pure water, and then dried in a vacuum oven at 60 °C for 24 h. Gas permeability measurements Gas permeability measurements were performed using a custom test chamber. The porous polymeric membranes were masked by first placing a section of the material on a 47-mm piece of adhesive-backed aluminium with a hole cut in the centre. The membrane/adhesive aluminium assembly was then attached to a 47-mm aluminium disk (1/16-inches thick) with a mating hole in the centre corresponding to the hole in the adhesive-backed aluminium, thus creating a sandwich. A thin layer of epoxy was placed on the interface between the porous membrane and the aluminium to seal the membrane completely and to ensure that the only available diffusion path would be through the membrane. The mounted membranes normally have an open area of 5–7 mm in diameter, which is exposed for gas permeability measurements. The thickness of the membrane was measured using high-resolution calipers. The membrane was then placed in the test chamber and evacuated to ~20 mTorr at which it remained overnight. Single gas permeability measurements were obtained by isolating the two parts of the chamber (the permeate and retentate) and introducing each gas to the retentate side until a pressure of 35 kPa was reached. The pressure rise on the permeate side was monitored using a 10-Torr Baratron gauge (MKS Instruments) and a data logging programme. After an initial delay time corresponding to the diffusion time through the membrane, the pressure in the permeate side rose linearly with time. From the slope of this pressure rise and the properties of the membrane, the permeability was calculated using the following equation (1): where V is the permeate volume, t is the membrane thickness, R is the gas constant, T is the absolute temperature, A is the membrane area, Δ p is the pressure difference across the membrane and dp/dt is the rate of gas pressure increase on the permeate side. The permselectivity for gas pairs (CO 2 –N 2 and O 2 –N 2 ) is simply the ratio of the single gas permeabilities. CO 2 /N 2 uptake Gas uptake measurements were obtained using a gravimetric microbalance (Hiden Isochema, IGA) that combines accurate computer control of pressure and temperature with high precision measurements of sample weight changes to acquire gas uptake isotherms. The sample was loaded into a quartz sample container and sealed in the stainless steel chamber. The sample was dried and degassed at a temperature of 60 °C and a vacuum pressure of 1 mbar for a minimum of 4 h before the dry mass was recorded. Mass measurements were then acquired at increasing CO 2 pressures up to ~1 atm, taking into account the buoyancy effect on the mass. The temperature of the sample was maintained using either a constant temperature recirculating water bath for the 298-K measurement or an ice bath for the 273-K measurement. High-resolution TEM imaging High-resolution TEM samples were imaged in a Carl Zeiss Libra 120 with an in-column energy filter. Experiments were performed at an acceleration voltage of 120 kV, an emission current of ~3 μA with a minimum dose condition to eliminate potential electron-induced sample damage. Nevertheless, the polymer samples show remarkable beam resistance. How to cite this article: Qiao, Z.-A. et al. Polymeric molecular sieve membranes via in situ cross-linking of non-porous polymer membrane templates. Nat. Commun. 5:3705 doi: 10.1038/ncomms4705 (2014).